Direct observation of ultrafast long-range charge separation at polymer–fullerene heterojunctions In polymeric semiconductors, charge carriers are polarons, which means that the excess charge deforms the molecular structure of the polymer chain that hosts it. This results in distinctive signatures in the vibrational modes of the polymer. Here, we probe polaron photogeneration dynamics at polymer:fullerene heterojunctions by monitoring its time-resolved resonance-Raman spectrum following ultrafast photoexcitation. We conclude that polarons emerge within 300 fs. Surprisingly, further structural evolution on ≲ 50-ps timescales is modest, indicating that the polymer conformation hosting nascent polarons is not significantly different from that near equilibrium. We interpret this as suggestive that charges are free from their mutual Coulomb potential because we would expect rich vibrational dynamics associated with charge-pair relaxation. We address current debates on the photocarrier generation mechanism at molecular heterojunctions, and our work is, to our knowledge, the first direct probe of molecular conformation dynamics during this fundamentally important process in these materials. In photovoltaic diodes based on blends of polymeric semiconductors and fullerene derivatives, photocurrent generation requires charge separation, with photoinduced electron transfer as an early step. From a semiconductor perspective, the electronic structure of the two materials define a type-II heterojunction, providing sufficient driving force to dissociate highly bound excitons on the polymer [1] . In spite of important progress to optimize the solar power conversion efficiency in polymer solar cells, the mechanism for the evolution from the non-equilibrium primary photoexcitation (the unrelaxed exciton on a polymer chain immediately after light absorption) to photocarriers (unbound charges) is not resolved and is currently the subject of vivid debate. Earlier studies of all-polymer donor:acceptor blends by Morteani et al. [2] concluded that an intermediate step between intrachain excitons and free charges is charge separation into Coulomb-bound electron-hole pairs, which we will refer to as charge-transfer states (CT), emphasizing that the electron and hole are mutually bound across the interface. After this initial step, the CT state can either branch directly to free charges or relax to an excitonic state bound at the interface between the donor and acceptor materials, a state termed charge-transfer excitons (CTX). Others also reported this branching behaviour in polymer:fullerene blends [3] , [4] . Later reports indicated that initial charge separation to CT states occurs on ≤100-fs timescales [5] , [6] . Furthermore, Jailaubekov et al. [7] concluded that at molecular-semiconductor heterojunctions, CT states must produce photocarriers on timescales faster than ∼ 1 ps if this process is to be competitive against relaxation to the CTX state, as the binding energy of CTX is typically ∼ 10 k B T at room temperature [8] , [9] , rendering photocarrier generation from those states energetically unlikely in principle. Nevertheless, these relaxed CTX can be ‘pushed’ with an infrared optical pulse resonant with an intraband polaronic optical transition to promote them to a delocalized, near-conduction-edge state that can then dissociate into charge carriers, thus enhancing photocurrent [10] . However, Lee et al. [11] and more recently Vandewal et al. [12] have argued that relaxed CTX states, when excited directly, are in fact the photocurrent precursors in many if not most polymer:fullerene systems. The contemporary literature therefore reflects disagreement on whether rapid dissociation of non-equilibrium intrachain excitons or CT excitons is a significant pathway towards photocurrent generation in polymer diodes. The seemingly conflicting scenarios are all based on probing population dynamics by time-resolved spectroscopies, or directly probing photocurrent internal quantum efficiency spectra in conjunction with steady-state absorption and luminescence measurements, both of which provide limited direct mechanistic insight into photocarrier generation dynamics. In this work, we exploit femtosecond stimulated Raman spectroscopy (FSRS), an ultrafast optical probe that is simultaneously sensitive to molecular-structure and electronic-population (excitons, polarons) dynamics. 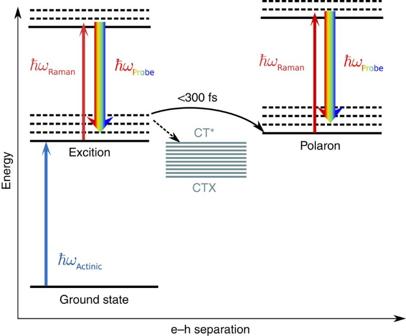Figure 1: Schematic diagram of the photophysics reported in this article. Shown are the role of the actinic, Raman and probe pulses in generating the FSRS signal. The intrachain exciton, hole–polaron, CT and CTX states, discussed in the article, are depicted. Our choice of Raman photon energy, which is resonant with an excited-state absorption, probes selectively photoexcitations on the donor polymer. Note that formally the depicted excitonic (and polaronic) vibronic levels are vibronic bands in polymeric semiconductors (see ref.60). Figure 1 depicts how this optical probe measures time-resolved resonance-Raman signatures of excitons and polarons in the system discussed here: after selective photoexcitation of the polymer with an ‘actinic’ ultrashort pulse, a combination of a ‘Raman’ picosecond pulse and a femtosecond broadband ‘probe’ pulse generates excited-state stimulated resonance-Raman signal as a function of delay between actinic and probe pulses. This spectroscopy is therefore an intricate probe of charge photogeneration dynamics since charges in polymeric semiconductors are polaronic, in which the charge distorts the polymer backbone surrounding it, producing unambiguous molecular vibrational signatures. Figure 1: Schematic diagram of the photophysics reported in this article. Shown are the role of the actinic, Raman and probe pulses in generating the FSRS signal. The intrachain exciton, hole–polaron, CT and CTX states, discussed in the article, are depicted. Our choice of Raman photon energy, which is resonant with an excited-state absorption, probes selectively photoexcitations on the donor polymer. Note that formally the depicted excitonic (and polaronic) vibronic levels are vibronic bands in polymeric semiconductors (see ref. 60 ). Full size image Although ultrafast solvatochromism-assisted vibrational spectroscopy has been used to study charge dynamics in fullerene aggregates [13] , our work is to our knowledge the first direct time-resolved vibrational probe of polaron formation dynamics on polymers at polymer:fullerene heterojunctions. We find that by optical excitation of the lowest (π,π*) optical transition in the polymer, clear polaronic signatures are present within the early-time evolution of the photoexcitation, on ≲ 300-fs timescales, in a benchmark polymer:fullerene blend, depicted as a direct production of polarons in Fig. 1 . Surprisingly, we observe limited vibrational relaxation following this ultrafast process, indicating little structural changes occuring on time windows spanning up to 50 ps, which we interpret as indicative of holes on the polymer that are sufficiently far from their electron counterparts such that they are free of their Coulomb potential. We interpret these surprising results as suggestive that in this system, which produces among the highest efficiency solar cells, intermediate CT state (Coulomb-bound electron-hole) pairs are not prerequisite species for photocarriers because vibrational signatures of polarons emerge at a faster rate than exciton relaxation by at least one order of magnitude. Based on this premise, we conclude that ultrafast dissociation of non-equilibrium photoexcitations is a significant process in this system. Femtosecond stimulated Raman spectroscopy We implement FSRS to characterize the molecular structural dynamics in a model semiconductor copolymer used in efficient solar cells during charge transfer to a fullerene acceptor in the solid state [14] . FSRS measures the transient stimulated resonance-Raman spectrum of the photoexcited species by preparing the polymer in its excited state with a short actinic pulse ( ∼ 50 fs, 560 nm), and then probing the evolution of the stimulated Raman spectrum with a pair of pulses: a Raman pump pulse resonant with a photoinduced absorption of interest (1.5 ps, 900 nm) and a short ( ∼ 50 fs) broadband probe pulse to generate the excited-state stimulated Raman spectrum of the transient species at various delay times between the actinic and Raman-pump/probe pulses. The time resolution of ultrafast FSRS stems then from the ability to precisely initiate the vibrational coherence in a molecular system from the two laser pulses that gives rise to the measured signals. FSRS thus permits measurement of the time-resolved, excited-state resonance-Raman spectrum over relevant timescales over which molecular conformational changes take place [15] . We collect concomitantly transient absorption spectra by monitoring the differential transmission of the broadband probe pulse induced by the actinic pulse (that is, by measuring the signal without the Raman pump pulse). In our studies, we apply this technique on poly(N-9′-heptadecanyl-2,7-carbazole-alt-5,5-(4′,7′-di-2-thienyl-2′,1′,3′-benzothiadiazole) (PCDTBT), which is a carefully engineered ‘push–pull' material system for solar cells, with reported solar power conversion efficiency of 6 (ref. 16 ) to 7.2% (ref. 17 ), unusually high internal quantum efficiency approaching 100% (ref. 16 ), and reported ultrafast charge separation in fullerene blends [5] , [18] , such as fullerene derivative [6,6]-phenyl-C 61 butyric acid methyl ester (PCBM). Polaronic signatures Unequivocal identification of polarons in PCDTBT ( Fig. 2a ) requires knowledge of the spectral signatures of its cations. To measure them, we oxidized a neat polymer film, that is a film composed only of the polymer donor material, with FeCl 3 , which is known to dope polycarbazoles [19] . The ground-state absorption spectrum of the doped film ( Fig. 2b ) features a low-energy absorption band centred around 1.7 eV, which has been assigned to cations in previous doping studies [19] . This absorption band in the doped film corresponds to the ‘interband’ polaronic transition [20] . It matches closely the transient absorption band of the PCDTBT:PCBM blend in the 1.2–2.0 eV region ( Fig. 2c ), which reinforces the previous assignment of this photoinduced absorption band to polarons [5] , [18] . Excitation of the doped PCDTBT film within the low-energy band at 830 nm (1.49 eV) provides thus the resonance-Raman spectrum of the polaron ( Fig. 2d , grey), which is the vibrational fingerprint of that photoexcitation on PCDTBT. 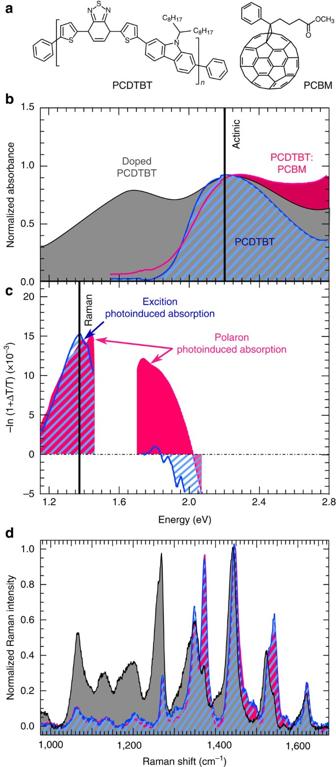Figure 2: Ground- and excited-state absorption and Raman spectra of films of neat PCDTBT and PCDTBT:PCBM. (a) Structure of PCDTBT (left) and PCBM (right). (b) Absorption spectra of neat PCDTBT (blue), PCDTBT:PCBM (pink) and doped PCDTBT (grey) films. (c) Transient absorption spectra of the same samples as in part (a). The broad gap around 1.55 eV (800 nm) results from a notch filter used to remove residual laser fundamental light. (d) Resonance-Raman spectra of the same samples as ina. The wavelength of the actinic (the femtosecond pump) and Raman (picosecond pump) pulses are indicated by vertical lines inbandc. Figure 2d also shows the resonance-Raman spectra of neat PCDTBT and PCDTBT:PCBM, excited at 514 nm (2.30 eV). To aid with assignment of these peaks, we calculate Raman frequencies of the ground, excited and cationic states of the PCDTBT dimer in vacuum using density-functional theory (DFT) and time-dependent DFT (TDDFT) utilizing the B3LYP functional. We then identified the modes of the measured Raman peaks by comparing them to the frequency of the bands in the theoretical Raman spectrum ( Supplementary Fig. 1 ) and to a published resonance-Raman study of PCDTBT [21] . These assignments are summarized in Tables 1 and 2 . We note that a combined electron paramagnetic resonance and DFT report points out that the degree of localization of polarons is influenced by the presence of counterions in doped films [22] , which is likely to influence the details of the resonance Raman signatures assigned to polarons in the doped PCDTBT film compared with polarons in the pristine blend. Nevertheless, the spectra reported in Fig. 2d represent an important starting point for our assignment of FSRS spectra below. Figure 2: Ground- and excited-state absorption and Raman spectra of films of neat PCDTBT and PCDTBT:PCBM. ( a ) Structure of PCDTBT (left) and PCBM (right). ( b ) Absorption spectra of neat PCDTBT (blue), PCDTBT:PCBM (pink) and doped PCDTBT (grey) films. ( c ) Transient absorption spectra of the same samples as in part ( a ). The broad gap around 1.55 eV (800 nm) results from a notch filter used to remove residual laser fundamental light. ( d ) Resonance-Raman spectra of the same samples as in a . The wavelength of the actinic (the femtosecond pump) and Raman (picosecond pump) pulses are indicated by vertical lines in b and c . Full size image Table 1 Neat and pristine (undoped, as cast) PCDTBT film spontaneous resonance Raman and FSRS shifts. Full size table The differences in intensities of the cation resonance-Raman spectrum with respect to that of the pristine (as-cast) film, consisting of neutral polymer chains, reveal differences in the geometric distortion between the ground and the resonant-electronic states along the normal coordinate for each mode. In particular, the Raman spectrum on resonance with the polaronic transition shows a marked enhancement of bands corresponding to carbazole and thiophene local modes between 1,000 and 1,200 cm −1 , as well as in benzothiadiazole and carbazole bands at 1,268 and 1,349 cm −1 , which are more delocalized ( Supplementary Fig. 2 ). This is consistent with the electronic density shift between the highest occupied molecular orbital (HOMO) and the lowest unoccupied molecular orbital (LUMO) of the charged polymer, which affects mainly the carbazole and the thiophene units ( Supplementary Fig. 3 ). On the other hand, the resonance-Raman spectra of PCDTBT and PCDTBT:PCBM exhibit strong enhancement of modes predominantly involving motion of the benzothiadiazole unit at 1,370 and 1,540 cm −1 . This is consistent with the electronic density shift between the HOMO and the LUMO of the neutral polymer, which involves the localization of the wavefunction on the thiophene–benzothiadiazole–thiophene unit ( Supplementary Fig. 4 ). Excited-state Raman dynamics in the blend The temporal evolution of the FSRS spectrum of a PCDTBT:PCBM film is illustrated in Fig. 3a,b (see Supplementary Figs 5 and 6 for FSRS spectra at all recorded time delays). We use a Raman pump pulse at 900 nm (1.38 eV) to be on resonance with the low-energy part of the polaron optical absorption spectrum, and thus these figures represent the temporal evolution of the stimulated resonance-Raman spectrum of the photoinduced polarons in PCDTBT:PCBM heterojunctions. We note the striking similarity of the transient FSRS spectra with the steady-state, spontaneous resonance-Raman spectrum of the doped PCDTBT film, confirming that we are probing hole polarons directly on the PCDTBT backbone. The characteristic bands of this polaronic signature readily follow the ultrashort actinic pulse ( Supplementary Fig. 7 ), in particular the 1,357 cm −1 band that is absent from the FSRS neat PCDTBT spectrum at any delay time ( Fig. 3c ) and the 1,260 cm −1 band that is present in the latter FSRS spectrum with a low intensity. The nature and timescale of molecular changes that FSRS is able to follow has been the subject of recent discussions [23] , [24] , [25] . This is because at early times, after electronic excitation, the molecular system may not have equilibrated and its vibrational signatures are changing during this evolutionary phase [23] . FSRS signals do not represent instantaneous frequencies present at the sample when the probe pulse (the white-light continuum) arrives. The FSRS signal arises via the initiation of a vibrational coherence as it interacts with the Raman pump pulse and therefore the signals we observe develop over the vibrational dephasing time [24] . The temporal resolution of FSRS is provided by the ability to use a femtosecond actinic pulse to photoexcite the sample followed by precisely generating the vibrational coherence leading to the FSRS signals. The cross correlation between the two femtosecond pulses is well defined and small, here 100 fs. However, the overall spectral resolution is determined by both the excited vibrational coherence free induction decay (typically 1–3 ps) and the Raman pump pulse duration. That is the frequency linewidth of the vibrational mode being dictated by the Fourier transform of the coherence decay convoluted with the Raman pump pulse duration provide a time and bandwidth product that does not violate the uncertainty principle, Δ ω Δ t ≤1. The ability of FSRS to capture frequency changes occurring on timescales faster than the dephasing time is due to the detection method, because signals are generated by the interference of the two optical fields (a form of heterodyne detection) [15] ; however, in such cases the spectral lines would be consequently broadened. With such a method, at very early times, as coherences between the optically applied field and the molecular eigenstates are lost due to both electronic and configurational changes, ‘derivative' line shapes can be observed as spectral features. These can be deconvoluted to reveal time-dependent molecular frequencies as recently demonstrated for the case of rhodopsin by McCamant [24] . In our FSRS spectra, ‘derivative’ line shapes are only observed at the earliest time delays, indicating that the establishment of product modes following the electronic excitation and charge transfer is extremely rapid. Furthermore, the fact that we observe Raman spectra that do not change above a few-hundred-femtosecond time delays, and that the spectra are extremely similar to those of the product states, has to be taken as evidence that we are observing a molecular state that is representative of the product state, namely the PCDTBT cation, and this confirms that the CT reaction is occurring well within the few-hundred-femtosecond timescale. The structurally sensitive method of FSRS thus establishes unambiguously that polarons in PCDTBT:PCBM blends are created over one order of magnitude faster than electron density transfer in the neat polymer (see below). 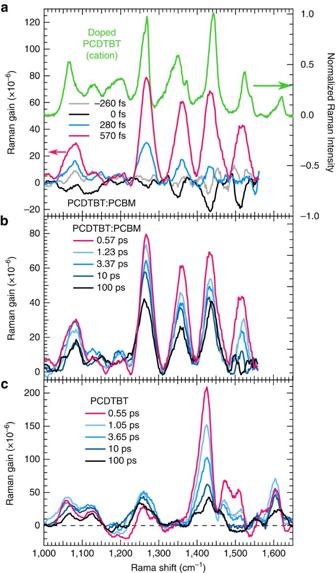Figure 3: FSRS spectra of PCDTBT:PCBM and neat PCDTBT. Shown are femtosecond stimulated Raman spectra of (a,b) PCDTBT: PCBM and (c) neat PCDTBT films to illustrate structural relaxation over a 100-ps time window. Spontaneous resonance-Raman of doped PCDTBT (green) is also shown inafor comparison. Figure 3: FSRS spectra of PCDTBT:PCBM and neat PCDTBT. Shown are femtosecond stimulated Raman spectra of ( a , b ) PCDTBT: PCBM and ( c ) neat PCDTBT films to illustrate structural relaxation over a 100-ps time window. Spontaneous resonance-Raman of doped PCDTBT (green) is also shown in a for comparison. Full size image The structural distortion imposed on the polymer through the generation of the radical cation can be characterized through the frequency shifts in the FSRS bands in the spectrum of the blend film (see also Supplementary Note 1 ). A significant upshift of 20 cm −1 is observed for the 1,064 cm −1 mode involving the thiophene C–H bend and C=C stretch, implying an increase in bond order of the latter bond associated with the transition to a quinoidal state. This is supported by the 13 cm −1 decrease in the frequency of the 1,444 cm −1 band associated with the other two C=C bonds in thiophene, as well as increase in the frequency of C=C stretching carbazole modes, demonstrating the alternation of single double bonds. While the differences in the Raman spectrum between the ground and excited states reflect differences in structure between the ground and excited electronic states, the small changes in the Raman spectrum of the excited state observed as a function of time indicate that any structural changes occurring during electronic and vibrational relaxation are small. Indeed, the overall shape of the FSRS spectrum of PCDTBT:PCBM at >500-fs timescales is essentially constant and decays with the population dynamics ( Fig. 4a and Supplementary Fig. 7 ), with the exception of the carbazole mode at 1,513 cm −1 whose dynamics will be discussed later in this article. Since the spectral signature of polarons emerges in the relaxed structure form at timescales earlier than what we would expect from structural reorganization, this hints that the conformation of the polymer emerging from the Franck–Condon region is already close to the relaxed hole conformation. 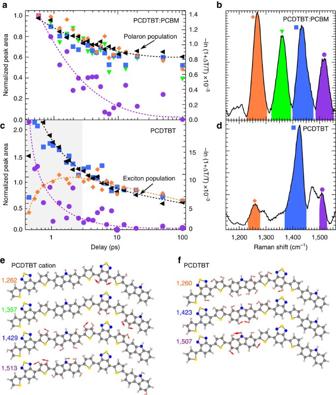Figure 4: Comparison of FSRS and transient absorption dynamics. Shown are the dynamics of the stimulated Raman peak areas (extracted by Gaussian curve fit) and the excited species population in (a) PCDTBT:PCBM and (c) PCDTBT films. The analysed FSRS peaks for the neat material and the blend, along with the symbol key for the time-resolved data shown inaandc, are shown inbandd, respectively. The data are normalized at 4 ps foraand at 0.6 ps inc. The dotted lines inaandcare meant as a guide to the eye. Vector diagrams showing vibrational motion associated with the corresponding analysed peaks in a dimer of PCDTBT, determined byab initiocalculations, are displayed for the cation (e) and the neutral molecule (f). Animations of those vibrational modes can be viewed asSupplementary Movies 1–7. Figure 4: Comparison of FSRS and transient absorption dynamics. Shown are the dynamics of the stimulated Raman peak areas (extracted by Gaussian curve fit) and the excited species population in ( a ) PCDTBT:PCBM and ( c ) PCDTBT films. The analysed FSRS peaks for the neat material and the blend, along with the symbol key for the time-resolved data shown in a and c , are shown in b and d , respectively. The data are normalized at 4 ps for a and at 0.6 ps in c . The dotted lines in a and c are meant as a guide to the eye. Vector diagrams showing vibrational motion associated with the corresponding analysed peaks in a dimer of PCDTBT, determined by ab initio calculations, are displayed for the cation ( e ) and the neutral molecule ( f ). Animations of those vibrational modes can be viewed as Supplementary Movies 1–7 . Full size image Excited-state Raman dynamics in the neat film Having established that polarons appear on ultrafast timescales in PCDTBT:PCBM blends, we address whether they are readily observable in the neat polymer as well. The FSRS spectra of neat PCDTBT, reported in Fig. 3c , do not display polaronic signatures, excluding that species as a direct photoexcitation on the neat polymer on timescales shorter than 100 ps. In particular, the 1,357 cm −1 band is absent, and the relative intensity of the 1,260 cm −1 band with respect to the 1,429 cm −1 band is at least four times lower at 0.5 ps. As the excitation decays, we do not observe the rise of the characteristic 1,357 cm −1 band, indicating that there is no conversion of the initial excitation into polarons at later times. Therefore, polarons are not a dominant primary photoexcitation in neat PCDTBT. We thus assign the observed FSRS spectra in the neat PCDTBT film to intrachain singlet excitons as primary photoexcitations. Indeed, Etzold et al. [18] assigned the photoinduced transient absorption band in neat PCDTBT, centred at the energy we use for our Raman pump (1.38 eV), to singlet excitons, while triplets were argued to form on timescales much longer than those explored in the present experiment [21] . In addition, the calculated exciton Raman spectral line shape in PCDTBT from our TDDFT calculations is in remarkable agreement with the experimental data ( Supplementary Fig. 1 ), which further supports our assignments. These direct structural measurements have important implications on our understanding of ‘push–pull’ co-polymers, which comprise electron-rich and electron-poor moieties within the polymer repeat unit. Indeed, a hypothesis to rationalize the generally high solar power-conversion efficiency of this class of co-polymers would be that they readily form loosely bound polaron pairs upon photoexcitation, without the aid of a fullerene acceptor [20] , [26] . The evidence presented here in favour of the singlet exciton contradicts this hypothesis. We underline that according to our calculations and other work [21] , [27] , the singlet exciton exhibits some degree of CT-like character. However, we insist that this picture is distinct from the loosely bound polaron pairs hypothetized for similar ‘push–pull’ co-polymers as noted above. The evolution of the FSRS spectral line shape in neat PCDTBT is complex, but is consistent with transfer of electron density to the acceptor unit on the polymer (TBT) on a picosecond timescale. To appreciate the evolution of individual modes, we extract their kinetics by fitting FSRS peaks with a Gaussian curve and report their area as a function of time on Fig. 4c , comparing them with population dynamics extracted from transient absorption measurements probed at 1.2 eV (1,035 nm). The most intense FSRS peak at 1,429 cm −1 , comprising mainly thiophene C=C stretching and carbazole C–N–C bending/C–C stretching follows the exciton population dynamics after 1 ps. However, other bands deviate significantly from population dynamics. Specifically, the 1,507 cm −1 peak decays to 25% of its initial intensity within 3 ps, while the 1,260 cm −1 band grows on a similar timescale. The 1,507 cm −1 band is a carbazole mode not visible in the ground state of neutral PCDTBT. However, our TDDFT calculations reveal that coupling with neighbouring thiophenes activates this mode. The 1,260 cm −1 band is a delocalized mode characterized by C–H in-plane bending and C=C stretching in the BT phenyl ring along with C–N stretching in the thiadiazole ring in addition to carbazole and thiophene motion, and hence is sensitive to changes in electronic density on the acceptor unit. A slow increase in intensity is also observed in other modes, such as the 1,057 cm −1 thiophene C–H bending mode. The evidence provided by FSRS thus helps draw a picture of the exciton evolution following photoexcitation to the Franck–Condon region, where the wavefunction is initially delocalized along the polymer chain [28] . The rapid decay of the 1,507 cm −1 mode indicates that initial enhancement is lost either due to the loss of coupling as predicted by the TDDFT calculations and/or changes to the Raman cross section upon shifting of electron density from carbazole to the benzothiadiazole acceptor. This shift in electronic density is evidenced by the growing intensity of the 1,260 cm −1 band. Transfer of the electronic density to the benzothiadiazole and thiophenes on a few-picosecond timescale is consistent with the calculated localization of the electronic density in the LUMO ( Supplementary Fig. 4 ), and is in general agreement with the 1-to-10-ps timescale reported for exciton dynamics in conjugated polymers [29] , [30] . Therefore, the rich dynamics that develop in this excitonic system probed by FSRS reflect the dynamics of electron density flow in the polymer on a much slower timescale than the observed charge separation process in the blend system. FSRS dynamics We now return to a discussion of the FSRS dynamics displayed in Fig. 3a,b , in which we had pointed out that the overall shape of the FSRS spectrum of PCDTBT:PCBM at early times is comparable to that of the relaxed structure (100 ps and beyond) and decays with the population dynamics ( Fig. 4a and Supplementary Figs 7 and 8 ). As noted above, the only rapid FSRS dynamics that we observe involve the decay of the mode at 1,513 cm −1 ( Supplementary Fig. 9 ). In fact, the 1,200 cm −1 mode displays similar behaviour, though its modest intensity makes quantitative analysis challenging. Interestingly, what these two modes have in common is that their band intensity depends on the extent of the coupling between carbazole and its neighbouring thiophene. We can rationalize the decay dynamics of these modes by a dynamic decoupling of carbazole and thiophene, possibly arising from evolution of the dihedral angle between these moieties. We also note that although the 1,513 cm −1 mode decays rapidly, this decay is slower in the blend than for the 1,507 cm −1 mode in the neat film ( Fig. 3c ). This suggests that the mechanism in the blend is distinct from the excitonic behaviour in the neat film. Insight on the significance of those dynamics can be gained by considering previous work by Pensack et al. [13] focusing on a carboxyl spectator mode in PCBM using ultrafast solvatochromism-assisted vibrational spectroscopy. These authors proposed that vibrational energy originally in Franck–Condon active modes in a polymer:PCBM electron transfer reaction redistributes on a few-picosecond timescale into a distribution of vibrational modes including those involved in electron transport between PCBM molecules [13] . We speculate that the rapid relaxation of the 1,513 cm −1 mode could be related to mobile hole polarons as they move away from the interface. In contrast to the modest relaxation of the polymer backbone in the presence of nascent hole-polarons, the overall spectral shape of the FSRS spectrum of neat PCDTBT, hosting excitons as the dominant photoexcitation, evolves continuously during the first 100 ps after photoexcitation and probably beyond, which indicates that after the initial fast electron-density redistribution, a slower structural relaxation takes place. This indication would explain fluorescence up-conversion measurements on PCDTBT thin films, which show that the photoluminescence spectrum red shifts to its relaxed state within 200 ps (ref. 31 ). In particular, we observe red-shifting of the 1,260 and 1,471 cm −1 bands that correspond to benzothiadiazole and carbazole motion likely due to change in the bond order of the backbone in the thiophene–benzothiadiazole–thiophene unit, and shift of the electron density from the carbazole to the acceptor moiety, lengthening thus the carbazole C–C bonds ( Supplementary Fig. 4 ). On the other hand, the 1,429 cm −1 thiophene and carbazole band blue-shifts significantly between 50 and 100 ps, reflecting structural reorganization accompanied by vibrational relaxation on those timescales, involving possibly dihedral angle changes between the two units. Two key observations are presented in this paper. First, in PCDTBT:PCBM, ultrafast charge transfer happens before exciton relaxation dynamics on the few-picosecond timescale, as determined by the emergence of polaron resonance-Raman signatures on PCDTBT on timescales well within a few hundred femtoseconds. Second, once formed on sub-picosecond timescales, polaron resonance-Raman signatures do not undergo significant spectral shifts or changes in linewidth during the first 50 ps. The first result strongly indicates that electron transfer occurs before exciton relaxation following photoexcitation of PCDTBT blended with PCBM. We consider the nature of this prompt charge-separated excitation—Coulomb-bound electron-hole pair versus unbound charges with correspondingly large separation—by comparing to previous Raman studies on charge separation in solution as follows. In a previous FSRS study employed to follow the charge separation process of a non-covalent charge transfer complex in solution, Fujisawa et al. [32] observed that the frequencies of Raman modes remained constant throughout the process, and concluded that the Franck–Condon state had significant charge-separated character, which is a very similar scenario as presented here. Earlier work by Vauthey et al. [33] utilized time-resolved resonance-Raman spectroscopy with nanosecond resolution to follow the separation of a geminate ion pair into free ions in solution, and the authors distinguished between loosely bound charge pairs and separated ions invoking changes in the band frequencies. We thus expect that the FSRS spectrum of PCDTBT:PCBM is a very sensitive probe of the nature of the charged photoexcitation following initial charge separation and speculate that polarons, not CT excitons, are the photoproduct of such rapid dynamics, as we do not observe the dynamic signatures of separation of geminate pairs as observed by Vauthey et al. [33] This would imply that the corresponding electron on a PCBM phase, not detected by our FSRS measurements, must be separated over a sufficiently large distance on average in order for the polaron on the polymer backbone to not evolve under the resulting Coulomb potential on subnanosecond timescales, as evolution within such potential would result in evolution of the FSRS spectral line shape. In the dielectric environment defined by this class of materials, this separation must be in the order of several nanometres. In fact, Gélinas et al. [34] have analysed signatures of a transient Stark effect in the photobleach component of a transient absorption measurement in molecular donor blends with PCBM, and have concluded that over ∼ 40 fs the average electron-hole separation evolves to several nanometres, supporting our conjecture. Other transient absorption measurements on PCDTBT:PCBM or related donor materials also argue direct free-polaron generation on <100 fs timescales [6] , [5] , [35] , [36] . Such rapid, long-range charge transfer can be rationalized by exciton delocalization phenomena [28] , [37] , which can generally persist over sufficiently long timescales to play a role in the charge separation dynamics of interest in this work. Understanding the mechanism of ultrafast charge separation is important, as it was demonstrated that even when electronic alignments are unfavourable to charge separation (for example, in the presence of triplets), ultrafast kinetics can dominate and lead to very high internal quantum efficiencies [38] . Golden-rule formalisms applied to molecular electron transfer between localized asymptotic states cannot generally describe such rapid dynamics; however, when formulated in a delocalized basis set, such rapid dynamics can be readily described [39] . Along these lines, Savoie et al. [40] recently argued that resonant coupling of singlet excitons on the polymer to a high-energy manifold of fullerene band-like electronic states is what leads to efficient charge generation in systems such as PCDTBT:PCBM, bypassing localized CT states. Under this scenario, it is the high density of acceptor states in fullerene crystalline clusters that is responsible for direct photocarrier generation. Another possible mechanism under which ultrafast electron transfer can occur is bath-induced coupling of asymptotic eigenstates of the system [41] . In this mechanism, the vertical, non-equilibrium exciton state transfers by resonant tunnelling to a delocalized CT state induced by a dynamic coupling due to common zero-point fluctuations within a vibrational noise spectrum of the system. Indeed, such spectacularly rapid charge separation points strongly to quantum coherence dynamics, which are correlated to the dynamics of the molecular lattice [42] , and has been argued to play a key role in energy transfer dynamics in biological systems [43] . Either of these two mechanisms permit exciton separation over timescales that are much shorter than those in which a Marcus-theory description of ultrafast electron transfer is valid. Our second observation concerning the limited evolution of the Raman spectrum after polaron formation is surprising, since polaronic relaxation following ultrafast charge transfer is generally expected in these polymers composed of such complex repeat units. We observe clearly from the change in the excited state frequencies compared with the ground state that the polymer structure changes upon polaron formation within 300 fs in PCDTBT:PCBM, but the subsequent structural evolution over 50 ps is very modest, which we interpret as a signature that the nascent hole is sufficiently far from the electron counterpart such that they are free from their mutual Coulomb potential. If the charge pair was Coulomb-bound, we would expect evolution of the polaron vibrational signatures as the two charges relax within their attractive potential. While we cannot formally rule out that in PCDTBT:PCBM in the solid state the excited-state resonance-Raman spectrum characteristic in polarons should not be sensitive to the effective polarization evolution due to local electric fields resulting from Coulomb-bound polaron pairs, previous work on contact ion pairs in solution suggests that resonance-Raman probes are indeed very sensitive probes of such dynamics [33] , [44] , [45] . Particularly, a previous FSRS study concerning a coumarin:TiO 2 system also observed the absence of significant reorganization after charge formation [45] . Rapid charge separation is expected in that organic:inorganic hybrid system, since electron injection occurs into delocalized states in a conduction band of the inorganic nanostructure. The remaining positive charge on the dye therefore does not evolve under the influence of the electron potential. It is surprising that this seems to occur in PCDTBT:PCBM as well, given that such delocalized states in acceptor molecular aggregates are not expected a priori . These modes, that do not evolve after the initial charge transfer, are sensitive to the structure of the polymer, as exemplified by the frequency shifts of the modes between the ground and the polaronic state, which is of quinoidal structure, and also exemplified by the dynamics of the frequency shift of the main FSRS band in different solvents ( Supplementary Fig. 10 ). Regarding the modest structural evolution on the polymer, we note that Österbacka et al. [46] concluded that an increase in polymer chain stiffness is related to a smaller polaron relaxation energy. In a different vein, Coffey et al. [47] have suggested that a key route for improving future excitonic solar cells might be to reduce the reorganization energy inherent to photoinduced electron transfer. Indeed, we propose that correlating reorganization dynamics with macroscopic optoelectronic parameters will enable a fundamental understanding of the critical factors that lead to efficient photovoltaic systems at a molecular level. The modest polaron relaxation in PCDTBT:PCBM is an intriguing result, and one that opens a new door to understanding of the differences between material systems that produce efficient solar cells and those that should but do not perform as well, even if they obey the same ‘rational design’ principles based on empirical design rules relating device parameters (for example, open-circuit voltage and short-circuit photocurrent) to materials properties (for example, absorption spectral range, reduction potentials with respect to PCBM, and so on). Finally, we discuss that our two key observations indicate the possibility of parallel pathways for polaron formation in organic solar cells, as was also highlighted in the literature for P3HT:PCBM. Sheng et al. [48] demonstrated that polarons in P3HT:PCBM are created through two different channels: a direct, ultrafast one-step process and a slower, two-step process involving the creation and the dissociation of CT states, while Aryanpour et al. [49] applied a Coulomb-correlated Hamiltonian to find that fully separated charge-pairs are not a direct photoexcitation in polymer:fullerene heterojunctions. These two works would suggest that in some systems the rapid charge separation dynamics argued here are not observed. However, Gao and Grey [50] inferred that the dephasing of the vibronic coherence on ultrafast timescales does not depend on PCBM loading ratio in regiorandom P3HT:PCBM, indicating that ultrafast coupling to CT states is not significant. Therefore, because photocarriers are generated with high yield in that system, there must be a direct mechanism for their generation that must bypass CT intermediates. Similarly, the present work points strongly to direct photogeneration (that is, no CT intermediate) of unbound polarons in PCDTBT:PCBM, although it is also clear that CTX must form eventually in this system since in a previous publication we observed geminate recombination through CTX emission on nanosecond to microsecond timescales [51] . We note from our work, however, that the direct polaron-generation mechanism is operative on ultrafast timescales in PCDTBT:PCBM, with no forthright evidence of early involvement of intermediate CT states, while both channels may contribute to photocurrent in P3HT:PCBM. The degree of importance of the CT-state-mediated mechanism appears to be highly system-dependent. In ultrafast pump-push photocurrent measurements in polymer:PCBM photodiodes, Bakulin et al. [10] pumped the polymer with femtosecond pulses and then ‘pushed’ any Coulomb-bound charge pairs across the heterojunction with mid-infrared pulses resonant with sub-gap polaronic transitions. This promoted the charge pairs towards a delocalized state in which the charge pair could overcome their Coulomb binding and produce additional photocurrent. The degree to which Coulomb-bound charge pairs form following initial charge separation correlated with the degree to which additional photocurrent could be produced by pushing charges away from each other. Intriguingly, no additional photocurrent could be gained by application of the infrared push pulse in PCDTBT:PC 70 BM. This implies that a direct photocarrier mechanism is favoured in this system, which is in agreement with our conclusions that are based on a direct structural probe of polarons. If direct photocarrier generation is dominant in PCDTBT:PCBM and related efficient polymer systems [6] , avoiding the two-step process as is found in P3HT:PCBM [48] might be key in driving up efficiencies in solar cells by avoiding highly bound CTX states [9] , even if it is the case that these states are photocurrent precursors [12] . The conclusion that relaxation to bound charge pairs is limited in PCDTBT blends is the key observation that must be understood in order to better engineer polymers for solar-cell applications. In conclusion, we implement in this work FSRS on thin films of a photovoltaic-relevant polymer:fullerene heterostructure to reveal the structural dynamics of the polymer after photoexcitation, and assign the molecular origin of the observed features in transient absorption [5] and time-resolved photoluminescence [31] spectroscopies. Upon absorption in the lowest (π, π*) band at 2.21 eV (560 nm), ultrafast charge generation occurs within 300 fs to form a hole polaron on the polymer. The charge separation takes place before exciton localization (within 3 ps) in the neat film, while the exciton is far from vibrational equilibrium. Furthermore, vibrational relaxation of the resulting polaron on the polymer is modest over the first 100 ps, which we interpret as a signature that the hole is free from the Coulomb potential that the twin negative charge would impart. This mechanistic insight is key for future optimization of the efficiency of polymer:fullerene-based solar cells as it provides a window into the relationship between electronic dynamics and those of the polymer lattice involved in the conversion of excitons to photocarriers, which is of key importance for fundamental mechanistic understanding with molecular detail. Moreover, these conclusions are generally important in molecular photoexcitation because virtually every photochemical, photophysical or spectroscopic process in molecular materials involves coupled dynamics of electrons and the structure. Sample preparation PCDTBT ( M n =13,000 kg mol −1 ; M w =13,000 kg mol −1 ; PDI=2.3) was synthesized by S. Beaupré in the group of M. Leclerc [52] at Université Laval, as described elsewhere [52] and used as received. PCBM was purchased from Solenne (PCBM 60 , 99.5%, lot 15-05-12) and used as received. Thin films were wire-bar-coated at 100 °C on sapphire substrates (UQG Optics, 15-mm diameter, 1-mm thickness) using a bar with a channel width of 0.05 mm from solutions in 1,2-dichlorobenzene (HPLC grade, Alfa Aesar) of neat PCDTBT at a concentration of 8 mg ml −1 and PCDTBT:PCBM in a ratio of 1:4 at a concentration of 8 mg of polymer for 32 mg of PCBM in 1 ml. The polymer concentration was kept constant to preserve the required viscosity of the solutions to make the films. Morphologicial studies including X-ray, optical and thermal experiments on this material system can be found in Supplementary Figs 11 and 12 and Supplementary Note 2 . Spectroscopic methods Steady-state spontaneous Raman spectra were acquired with a Raman microscope (Renishaw inVia) with either 830- or 514-nm excitation. FSRS was performed at the Central Laser Facility of the Rutherford–Appleton Laboratory using the ULTRA set-up, a 10-kHz synchronized dual-arm femtosecond and picosecond laser system described elsewhere [53] . FSRS requires the generation of three pulses: the actinic pulse (560 nm, ∼ 50 fs), the Raman pulse (900 nm, 1.5 ps) and the broadband probe pulse ( ∼ 50 fs), which yields an experimental instrument response of ∼ 100 fs. These were generated using two custom titanium–sapphire amplifiers (Thales Laser) seeded from a single oscillator (20 fs, Femtolasers) to create synchronised femtosecond and picosecond outputs after compression, respectively. The femtosecond beam was split into two: one femtosecond beam pumped an optical parametric amplifier (Light Conversion TOPAS) to generate the actinic pulse, while the other femtosecond beam was focused onto a sapphire window to generate a white light continuum for the broad-band probe pulse. The 800-nm fundamental wavelength of the laser was then rejected from the white light continuum by a pair of notch filters (Kaiser Holographic notch plus) to avoid two-photon absorption in the sample. These notch filters are responsible for the gap at 800 nm in the transient absorption spectra presented in Fig. 2 . The picosecond beam was tuned to 900 nm by an optical parametric amplifier (Light Conversion TOPAS) and acted as the Raman pump pulse. The actinic and Raman beams were mechanically chopped at 5 and 2.5 kHz, respectively, while the probe beam was kept at the system repetition rate of 10 kHz. These different repetition rates create four different sequences of pulses, namely actinic-probe (01), Raman-probe (10), actinic-Raman-probe (11) and probe alone (00). The actinic-probe and probe alone sequences are used to obtain the transient absorption spectrum, while the FSRS spectra are obtained using a combination of those four sequences, as explained by Greetham et al. [53] Temporal dispersion of the pulses was minimized using reflective optics to transport beams to the sample. A linear motor drive translation stage (Newport) provided femtosecond to nanosecond pump-probe timing. The beams were focused onto the sample to typical beam diameters of 50 μm (probe beam) and 100 μm (actinic and Raman beams) set in a non-collinear geometry with an angle of 10° between the Raman and actinic beams and the probe. Samples were placed in a cold-finger cryostat (Janis Research Company) and kept under a dynamic vacuum (10 −6 mbar). Low temperatures were achieved by flowing liquid helium, reaching 100 and 180 K for the PCDTBT:PCBM and the neat PCDTBT films, respectively. The cryostat was rastered by a mechanical stage in the plane perpendicular to the beams to minimize cumulative photo-damage. After passing through the sample, the probe beam was collimated and focused into a spectrograph (0.25 m f/4 DK240, Spectral Products), then detected shot-by-shot using a custom high-rate-readout linear detector (Quantum Detectors). The spectra were averaged on a computer over 210,000 detected shots per spectrum for the neat PCDTBT film and 441,000 shots per spectrum for the PCDTBT:PCBM film. The spectra obtained were then smoothed using a feature-preserving Savitzky–Golay filter in MATLAB. The step size of the filter was small to avoid losing spectral accuracy. The FSRS spectra were baseline-corrected, using a polynomial fit to the broad background shape, preserving the FSRS peaks ( Supplementary Fig. 13 ). FSRS peak dynamics (peak area and centre frequency) were extracted by fitting a single Gaussian curve to individual peaks, or multiple Gaussian curves in areas of peak congestion. Computational methods All calculations were carried out within the framework of DFT [54] using Gaussian 03 and Gaussian 09 software [55] with the 6-311g(d) basis set [56] . The functional B3LYP (ref. 57 ) was used, which contains an empirically fitted percentage of exact-exchange for a better description of organic molecules. Other functionals were tested, such as CAM-B3LYP [58] , but the B3LYP was chosen due to a better description of the experimental vibrational spectrum of the ground state. All the optimization calculations were forced in a planar geometry, since the low-frequenecy torsion motion of the excited state threw the system out of the harmonic regime. Therefore, all torsion effects are not described by those calculations. While the ground-state and cation properties are calculated with DFT, the optically excited-state properties are obtained by applying TDDFT [59] . The new vibrational frequencies of each mode are obtained by fitting a parabola through nine single-point energy calculations around the energy minimum of the first singlet excited state, going from the minimum to the zero-point motion amplitude of the mode. This technique assumes that the effect on the frequency eigenvalues is limited to the first order, and that second-order effects of displacement eigenvectors can be neglected. The excited state intensities depend on the charge reorganization of the addition of an electron and a hole in our system, and they are approximated using the cation and anion ground state calculations. The ground-state mode is decomposed in the cation and anion vibrational modes, and a weighted average of all the intensities is taken accordingly, with equal weight between the cation and the anion, to obtain the new intensity. This technique neglects the effect of the interaction between the electron and the hole in the excited state. This effect is presumed to be small in the case of PCDTBT, since the description of the first singlet excited state after geometrical optimization is composed of 97% of the HOMO→LUMO transition. However, the new excited vibrational intensities must only be used to indicate the tendencies of the effects of the charge reorganization, and their quantitative significance is ambiguous. How to cite this article: Provencher, F. et al. Direct observation of ultrafast long-range charge separation at polymer–fullerene heterojunctions. Nat. Commun. 5:4288 doi: 10.1038/ncomms5288 (2014).